Unraveling oxygen vacancy site mechanism of Rh-doped RuO2catalyst for long-lasting acidic water oxidation Exploring durable electrocatalysts with high activity for oxygen evolution reaction (OER) in acidic media is of paramount importance for H 2 production via polymer electrolyte membrane electrolyzers, yet it remains urgently challenging. Herein, we report a synergistic strategy of Rh doping and surface oxygen vacancies to precisely regulate unconventional OER reaction path via the Ru–O–Rh active sites of Rh-RuO 2 , simultaneously boosting intrinsic activity and stability. The stabilized low-valent catalyst exhibits a remarkable performance, with an overpotential of 161 mV at 10 mA cm −2 and activity retention of 99.2% exceeding 700 h at 50 mA cm −2 . Quasi in situ/operando characterizations demonstrate the recurrence of reversible oxygen species under working potentials for enhanced activity and durability. It is theoretically revealed that Rh-RuO 2 passes through a more optimal reaction path of lattice oxygen mediated mechanism-oxygen vacancy site mechanism induced by the synergistic interaction of defects and Ru–O–Rh active sites with the rate-determining step of *O formation, breaking the barrier limitation (*OOH) of the traditional adsorption evolution mechanism. Oxygen evolution reaction (OER) plays an undoubtedly vital role in the energy conversion system, which involves hydrogen production through water electrolysis, CO 2 reduction to generate clean small molecule fuel, and the application of energy conversion devices such as metal-air batteries [1] , [2] , [3] , [4] . As a key half-reaction, OER needs higher energy to overcome the kinetic barrier due to the four-electron transfer reaction [5] , [6] , [7] . Compared with an alkaline medium, OER under an acidic electrolyte presents a higher reaction rate, fewer side reactions, and a more complete electrolytic cell system design during electrochemical water splitting, owing to the fully developed polymer electrolyte membrane (PEM) reduces gas crossover and provides high proton conductivity, and more importantly, hydronium ions have higher conductivity (350 S cm 2 mol −1 ) compared with hydroxide ions (198 S cm 2 mol −1 ) for large current density [8] , [9] . Therefore, it is voracious to exploit cost-effective alternative OER electrocatalysts with high activity and durability in an acidic medium. Currently, rutile-structured ruthenium (Ru) and iridium (Ir) oxides catalysts are widely used to improve the catalytic performance of acidic OER [10] , [11] , [12] . Notably, RuO 2 has higher activity and lower price than IrO 2 , being considered as a most potential acidic OER catalyst [13] , [14] . However, RuO 2 is limited by poor durability as a result of the collapse of active site structure and dissolution of Ru leading to deactivation under harsh acid conditions [15] , [16] , [17] , [18] . So far, it is generally accepted that the acidic OER mechanisms include the adsorption evolution mechanism (AEM) and the lattice oxygen mediated mechanism (LOM) [19] , [20] . The LOM can bypass the thermodynamic limitations of the typical AEM to enhance OER kinetics [21] , [22] . Recently, a series of LOM-based catalysts, including Si-SrCoO [21] , Zn 0.2 -Co 0.8 OOH [23] , and Ba 0.35 Sr 0.65 Co 0.8 Fe 0.2 O 3 -δ [24] , were explored to improve electrochemical performance toward OER in alkaline electrolytes by modulating the electronic structure of surface and interface. However, LOM is not as stable as AEM in acid because the lattice oxygen oxidation leads to severe surface remodeling of the catalyst, followed by dissolution in the electrolyte, affecting catalytic stability [8] , [25] . To achieve a balance between activity and stability, strategies of alloying [26] , [27] , defect engineering [28] , [29] , and heterogeneous element doping [30] , [31] are developed to promote rate-determining step (RDS) *OOH formation of AEM or prevent excessive oxidation of Ru-based materials into soluble Ru x+ (x > 4) derivatives (e.g., RuO 4 ) for LOM, simultaneously enhancing the activity and stability in acidic electrolyte. Among them, oxygen vacancies (O V ) in oxides can effectively change the coordination environment of the metal active center, expose more active sites, and enhance the intrinsic catalytic activity, which can be created by hydrogen reduction, high-temperature calcination, or low-valent element doping methods [32] , [33] . As we demonstrated previously, intrinsically defective RuO 2 via graphene oxide (GO) confined oxygenation strategy showed impressive OER activity but unfortunate stability [29] . Taken together, chemically stable O V and low-valent active center are crucial to stabilizing the catalyst, thereby maintaining the long-term stability of the acidic OER process. Inspired by the aforementioned design rationales, we herein develop Rh doping in RuO 2 lattice on graphene (Rh-RuO 2 /G) with ion-exchange adsorption strategy taking GO as the confined oxygenation template, yielding stable O V for compensating the effective negative charge of doped low-valent cations. More importantly, the rich O V surface sites also play key roles in the activity, including the O 2p band center is close to the Fermi level, which can accelerate charge transfer, while catalyst surface adsorption optimization achieves a lower reaction energy barrier and higher H 2 O activation rate [34] . In addition to the greatly enhanced catalytic activity, the doping of Rh provides stable O V for durable catalysis since it stabilizes the chemical coordination environment of the low-valent metal active sites for the OER process, proven by quasi in situ X-ray photoelectron spectroscopy (XPS) and ex-situ X-ray absorption fine structure (XAFS). Impressively, the enriched O V in the as-fabricated Rh-RuO 2 /G nanosheets exerted a decisive effect on OER activity and stability in acidic media. Specifically, the Rh-RuO 2 /G nanosheets display remarkable OER performance with an overpotential of 161 mV and 214 mV at a current density of 10 mA cm −2 ( η 10 ) and 100 mA cm −2 ( η 100 ), TOF of 1.74 s −1 at an overpotential of 300 mV, and long-durable stability of 700 h, suppressing most active OER electrocatalysts reported to date. Density functional theory (DFT) demonstrates that Rh-RuO 2 /G passes through a more optimal reaction path of the lattice oxygen mediated mechanism-oxygen vacancy site mechanism (LOM-OVSM) for activity, further elaboration of the stabilization mechanism. Particularly, the Rh-RuO 2 /G catalyst with excellent intrinsic structure also exhibits promising performance for Li-O 2 batteries, showing a small charge overpotential of 0.27 V and sustaining cyclability of 4500 h. Overall, the synergistic mechanism of Ru–O–Rh sites and stable O V shed new insight for rationally fabricating high-performance metal oxide catalysts. Synthesis and characterization of Rh-RuO 2 /G The Rh-RuO 2 /G catalyst was synthesized following the ion-adsorption approach [29] , as illustrated in Fig. 1a . 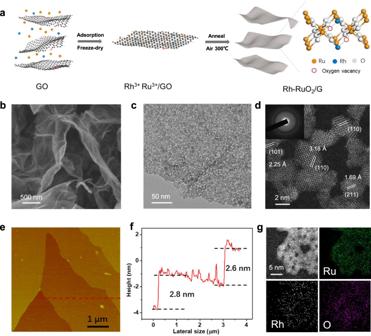Fig. 1: Synthesis and morphology characterization of Rh-RuO2/G nanosheets. aPreparation schematic.bSEM image.cTEM image.dHAADF-STEM image (inset shows the SEAD pattern).e,fAFM image (e) and corresponding height profiles (f).gElemental mapping analysis of Rh-RuO2/G. The Rh doping amount is 1.38 wt% in the RuO 2 matrix (Supplementary Table 1 ). Scanning electron microscopy (SEM, Fig. 1b ) and transmission electron microscopy (TEM, Fig. 1c ) images demonstrate the flexible laminar morphology of the as-prepared Rh-RuO 2 /G with smooth surfaces and evenly dispersed nanostructures. The average thickness of Rh-RuO 2 /G nanosheets is measured to be 2.7 nm, as identified by atomic force microscopy (AFM, Fig. 1e, f ), thereby exposing more inner layer atoms and providing effective active sites for catalytic reactions. The high-angle annular dark-field scanning TEM (HAADF-STEM) image in Fig. 1d shows the interconnecting small-size nanocrystals (≈2 nm) and lattice fringes corresponding to the (110), (101), and (211) planes for rutile-structured RuO 2 . Moreover, the selective electron diffraction (SAED) image indicates the polycrystalline nature of Rh-RuO 2 /G (inset in Fig. 1d ). Elemental mapping analysis (Fig. 1g ) confirms homogeneous distribution of Ru, Rh, O, and C signals throughout the entire nanosheet. Fig. 1: Synthesis and morphology characterization of Rh-RuO 2 /G nanosheets. a Preparation schematic. b SEM image. c TEM image. d HAADF-STEM image (inset shows the SEAD pattern). e , f AFM image ( e ) and corresponding height profiles ( f ). g Elemental mapping analysis of Rh-RuO 2 /G. Full size image The crystal structure of the as-obtained Rh-RuO 2 /G was validated by X-ray diffraction (XRD) pattern (Fig. 2a ), in which three prominent broadened diffraction peaks are well matched with the (110), (101), and (211) facets of rutile-structured RuO 2 (JCPDS no.40-1290), indicative of complete conversion of Ru 3+ into small RuO 2 . Electron paramagnetic resonance (EPR), as strong evidence for characterizing unpaired electrons, is used to explore the generation and variation of O V . Significantly, Rh-RuO 2 /G shows a significant EPR signal at g e = 2.003 (Supplementary Fig. 1 ) due to O V capturing unpaired electrons [35] . Raman spectrum shows the nanocrystalline nature of RuO 2 (Fig. 2b ), with three distinctive peaks centered at 516, 633, and 700 cm −1 corresponding to the E g , A 1g , and B 2g , respectively. After Rh doping, the peaks appear broadening and blue shift, signifying that local incorporation transforms the phonon vibration frequency by weakening symmetry and higher oxygen vacancy concentration promotes Ru–O vibration frequency [36] . It is noteworthy that the B 2g peak disappears in Rh-RuO 2 /G, which is attributed to the location of Rh(III) at the position of Ru(IV) sites in octahedral units by cations exchange rather than surface adsorption [37] , [38] . 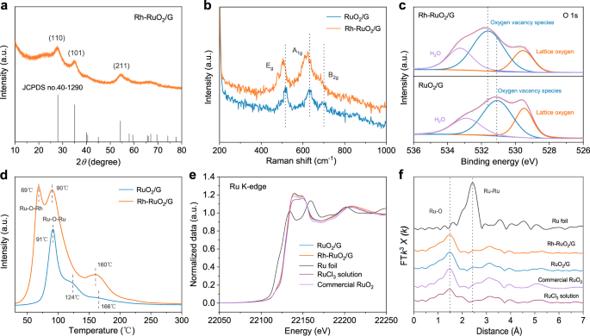Fig. 2: Compositional structure analysis of Rh-RuO2/G nanosheets. aXRD pattern of Rh-RuO2/G.bRaman spectra,cO 1sXPS spectra, anddH2-TPR spectra of Rh-RuO2/G and RuO2/G.eRu K-edge XANES spectra andfFourier transformed EXAFS spectra of Ru-edge for Rh-RuO2/G, RuO2/G, Ru foil, RuCl3solution, and commercial RuO2. Figure 2c compares the O 1s XPS to verify the defective structure. It can be seen that three well-fitted peaks are well deconvoluted into the lattice oxygen (Ru–O) at 529.5 eV, O V at 531.2 eV, and adsorbed water (H 2 O) at 533 eV, while the O V peaks for Rh-RuO 2 /G clearly shift to higher binding energy, proving the existence and chemical environment change of O V [39] . Significantly, the variation in the proportion of surface oxygen vacancy species and lattice oxygen (O V /O L ) is observed from 1.76 to 2.86 after doping, signifying an abundance of O V and thus excellent electronic capture and transfer properties of the nanosheets. It is understandable that O V are generated to maintain charge neutrality after exchanging a low oxidation state of Rh. The Ru 3p XPS spectrum (Supplementary Fig. 2a ) exhibits two predominant peaks located at 484.8 and 462.7 eV, slightly lower than the binding energy of Ru (IV) [40] . Similarly, the lower binding energy in the Rh 3d XPS spectrum (Supplementary Fig. 2b ) indicates the presence of low-valent Rh species, corresponding to 308.6 and 313.6 eV of anoxic rhodium oxides [41] . The H 2 temperature-programmed reduction (H 2 -TPR, Fig. 2d ) profile of RuO 2 /G exhibits a predominant peak located at 90 °C, corresponding to the conversion of Ru 4+ to metallic Ru, which is lower than the reduction temperature of commercial RuO 2 (213 °C) due to the small particle size [42] . The relatively weak peaks positioned at 100–200 °C can be ascribed to the variation in the particle sizes. In addition, Rh-RuO 2 /G shows a lower reduction peak at 69 °C as a result of the relatively weak asymmetric oxygen species (Ru–O–Rh), revealing the existence of an active center that requires further verification by DFT [43] , [44] . To further reveal the coordination structure and bond configurations of as-prepared Rh-RuO 2 /G, X-ray absorption spectroscopy (XAS) was employed to evaluate the valence state and coordination environment of Ru centers. The X-ray absorption near edge structure (XANES) of Ru K-edge region and the extended X-ray absorption fine structure measurements of Ru K-edge Fourier transformation (FT-EXAFS) are conducted with Ru foil, RuCl 3 solution, and commercial RuO 2 as references (Fig. 2e, f ). Figure 2e shows that the absorption threshold of Rh-RuO 2 /G lies between Ru foil and commercial RuO 2 , closing to RuCl 3 solution, visualizing the average valence state of Ru is between Ru(0) and Ru(IV) [45] , which is consistent with the XPS results. FT-EXAFS spectrum in Fig. 2f displays a main peak positioned at ~1.5 Å attributing to the backscattering of Ru–O in the first shell, while the Ru–Ru bond is at 2.4 Å [28] , [45] . The peak at 3.12 Å in Rh-RuO 2 /G originates from the backscattering of Ru–Ru and Ru–Rh in the second shell (Supplementary Fig. 4 ), exhibiting lower vibrational amplitudes than standard RuO 2 , which is ascribed to the small size of nanoparticles [13] , [46] . Besides, the Ru–O peak intensity of Rh-RuO 2 /G is slightly lower than standard RuO 2 , owing to the insufficient coordination of Ru. Compared with pure RuO 2 , the lower coordination number of 5.7 for Ru–O in Rh-RuO 2 /G is identified by EXAFS fitting results (Supplementary Table 2 ) as a result of O V , laying the foundation for theoretical computational modeling and mechanism analysis. Fig. 2: Compositional structure analysis of Rh-RuO 2 /G nanosheets. a XRD pattern of Rh-RuO 2 /G. b Raman spectra, c O 1s XPS spectra, and d H 2 -TPR spectra of Rh-RuO 2 /G and RuO 2 /G. e Ru K-edge XANES spectra and f Fourier transformed EXAFS spectra of Ru-edge for Rh-RuO 2 /G, RuO 2 /G, Ru foil, RuCl 3 solution, and commercial RuO 2 . Full size image Electrocatalysis of OER To demonstrate the catalytic ascendancy of rich O V with Rh doping, the OER performance of the Rh-RuO 2 /G catalyst was recorded in O 2 saturated 0.5 M H 2 SO 4 electrolyte. As shown by the linear sweep voltammetry (LSV) curves in Fig. 3a , the Rh-RuO 2 /G catalyst exhibits an η 10 of only 161 mV, which is lower than as-fabricated RuO 2 /G (203 mV) and commercial RuO 2 (297 mV), suggesting that the defects and Ru–O–Rh active center are conducive to acidic OER process with excellent performance. Moreover, our Rh-RuO 2 /G presents a significant small overpotential of η 100 = 214 mV (Fig. 3b ). Further, the Tafel slope of Rh-RuO 2 /G nanosheets is ≈45.8 mV dec −1 , smaller than those of RuO 2 /G (57.5 mV dec −1 ), and even the benchmark RuO 2 (60.4 mV dec −1 ) (Fig. 3c ). Such a low Tafel slope value signifies the fast kinetic merit of Rh-RuO 2 /G nanosheets for water oxidation. As depicted in Fig. 3d , the turnover frequencies (TOF) value corresponding to the intrinsic per site activity of the as-obtained Rh-RuO 2 /G is 1.74 O 2 s −1 at an overpotential of 300 mV, which is considerably higher than most reported catalysts [8] , [9] , [13] , [14] , [30] , [47] , [48] , [49] , [50] , [51] . Additionally, the electrochemical double-layer capacitance ( C dl ) values, extracted from cyclic voltammetry (CV, Supplementary Fig. 7 ), are closely associated with electrochemically active surface areas (ECSAs) of catalyst. Rh-RuO 2 /G displays noticeably larger C dl and ECSA values (110.6 mF cm −2 , 2765 cm 2 ) than RuO 2 /G (79.3 mF cm −2 , 1982.5 cm 2 ) and commercial RuO 2 (10.9 mF cm −2 , 272.5 cm 2 ) (Supplementary Fig. 6 ). It is indicated that Rh-RuO 2 /G nanosheets expose abundant active sites for facilitating OER activity. The electrochemical stability was evaluated by galvanostatic electrocatalysis. Obviously, Rh-RuO 2 /G maintains almost unchanged performance (99.2%) to the initial state for 700 h at a constant current density of 50 mA cm −2 , superior to RuO 2 /G and commercial RuO 2 (Fig. 3e ). The stability is further demonstrated by a long-term operation of 500 h at a higher current density of 100 mA cm −2 (Supplementary Fig. 8 ). Interpretably, the poor stability of RuO 2 /G originates from unrestricted O V and being vulnerable to destruction during the sustained OER process, while the doping of Rh creates a steady bulk O V structure and low-valent metal center for long-term durability. 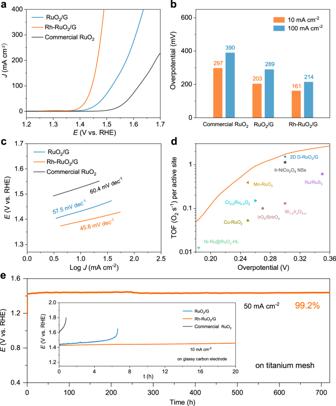Fig. 3: Electrocatalytic performance of Rh-RuO2/G, RuO2/G, and commercial RuO2catalysts in 0.5 M H2SO4solution with 95%iRcompensation. aLSV polarization curves.bOverpotentials at a current density of 10 mA cm−2and 100 mA cm−2.cTafel plots.dThe TOF curve of Rh-RuO2/G compared with reported representative catalysts.eThe galvanostatic curves at a current density of 10 mA cm−2and 50 mA cm−2. Therefore, our Rh-RuO 2 /G catalyst is one of the best acidic OER catalysts in terms of excellent overpotential and durability (Supplementary Table 3 ). To highlight the applicability for energy conversion, a two-electrode electrolyzer with Rh-RuO 2 /G as anode and Pt/C as cathode was performed for overall water splitting in acidic media. Remarkably, the polarization curve for water splitting exhibits a low cell voltage of 1.42 V at 10 mA cm −2 and maintains a pretty stable performance (Supplementary Fig. 9 ). Fig. 3: Electrocatalytic performance of Rh-RuO 2 /G, RuO 2 /G, and commercial RuO 2 catalysts in 0.5 M H 2 SO 4 solution with 95% iR compensation. a LSV polarization curves. b Overpotentials at a current density of 10 mA cm −2 and 100 mA cm −2 . c Tafel plots. d The TOF curve of Rh-RuO 2 /G compared with reported representative catalysts. e The galvanostatic curves at a current density of 10 mA cm −2 and 50 mA cm −2 . Full size image Structural analysis for enhanced activity and durability To probe the evolution of electronic structure at the surface of the catalysts, we carried out quasi in situ XPS studies to examine the potential-dependent oxidation of O 1s and Ru 3p 3/2 during the chronoamperometry test for OER, monitored by the analysis chamber of the in situ near ambient pressure XPS (NAP-XPS) system. 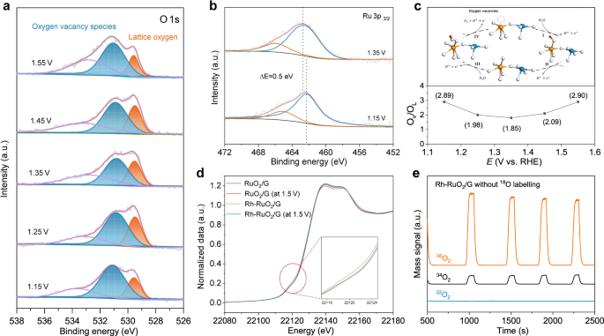Fig. 4: Quasi in situ NAP-XPS, ex-situ XAFS, and operando DEMS measurements probing dynamic evolution of electronic structure on Rh-RuO2/G catalyst during OER reaction. a,bThe quasi in situO 1s(a) andRu 3p3/2(b) XPS spectra recorded of the resultant Rh-RuO2/G during the multipotential steps.cVariation of OV/OLratio from quasi in situ XPS measurement.dEx-situ XANES spectra for Rh-RuO2/G and RuO2/G at 1.5 V for 8 h during OER. Inset: magnified pre-edge XANES region.eDEMS signals of36O2,34O2, and32O2for Rh-RuO2/G in H218O aqueous sulfuric acid electrolyte within four times of LSV at 1.1–1.9 V (vs. RHE). Figure 4a shows the variation in the proportion of surface oxygen vacancy species and lattice oxygen with the potential scanned from 1.15 to 1.55 V. A high ratio of O V /O L implies preferential adsorption of water at the intrinsic O V sites due to steric hindrance, which is closely connected with optimizing adsorption and desorption of intermediate oxygen species. Moreover, at higher potentials (1.55 V), the O V /O L ratio almost returns to the initial state (2.89), manifesting that O V regeneration is accompanied by the release of oxygen to endow the stabilization of the active site structure (Fig. 4c ) [52] . Similarly, the Ru 3p 3/2 peak position in Rh-RuO 2 /G shifts to higher binding energy ( ΔE = 0.5 eV) at 1.35 V (Fig. 4b ) since lower electron density around Ru atom after the lattice oxygen dominates. The phenomenon of cycling of reversible oxygen species demonstrates the priority of the LOM-OVSM, LOM-SMSM (the lattice oxygen mediated mechanism-single metal site mechanism). In order to further verify that lattice oxygen is not involved in OER, operando 18 O isotope labeling differential electrochemical mass spectrometry (DEMS) measurements were conducted. Figure 4e shows the main mass signals of 36 O 2 , followed by 34 O 2 and 32 O 2 , for the Rh-RuO 2 /G without 18 O-labeling during four times of LSV in H 2 18 O aqueous sulfuric acid electrolyte, where trace amounts of 34 O 2 product was attributed to the natural isotopic abundance of 18 O water～2 at.%. It is implied that the lattice oxygen atom is not participated in oxygen production, thereby excluding the traditional LOM. Consistently, a large number of 32 O 2 product was detected without any 36 O 2 for the 18 O-labeled Rh-RuO 2 /G catalyst in H 2 16 O aqueous sulfuric acid electrolyte (Supplementary Fig. 10 ). The quasi in situ XPS and DEMS results lay a foundation for theoretically simulating optimal reaction paths. Fig. 4: Quasi in situ NAP-XPS, ex-situ XAFS, and operando DEMS measurements probing dynamic evolution of electronic structure on Rh-RuO 2 /G catalyst during OER reaction. a , b The quasi in situ O 1s ( a ) and Ru 3p 3/2 ( b ) XPS spectra recorded of the resultant Rh-RuO 2 /G during the multipotential steps. c Variation of O V /O L ratio from quasi in situ XPS measurement. d Ex-situ XANES spectra for Rh-RuO 2 /G and RuO 2 /G at 1.5 V for 8 h during OER. Inset: magnified pre-edge XANES region. e DEMS signals of 36 O 2 , 34 O 2 , and 32 O 2 for Rh-RuO 2 /G in H 2 18 O aqueous sulfuric acid electrolyte within four times of LSV at 1.1–1.9 V (vs. RHE). Full size image Meanwhile, the stability of Rh-RuO 2 /G under working conditions was verified by operando Raman characterization techniques. As shown in Supplementary Fig. 11 , it is evidenced that the crystal structure keeps almost unchanged, as seen from the Raman vibrational displacement at the voltage of 1.05–1.9 V. To further explore the source of the stability difference, the local geometry evolution of Ru was observed by XANES under ex-situ conditions (Fig. 4d ). Compared with the stable absorption line of Rh-RuO 2 /G at initial and 1.5 V, RuO 2 /G depicts an obvious characteristic pre-edge 1s-4d transition after reaction (around 22120 eV), and the intensity of this shoulder peak is positively correlated with the unoccupied Ru 4d state [53] , [54] . It is disclosed that more electrons are transferred from 4d to nearby atoms, resulting in the increase of the average valence state of Ru, associated with additional oxygen species adsorption [6] , [55] . Therefore, it is inferred that the deactivation of RuO 2 /G is caused by the distortion of the coordination geometry and the weak change of the Ru oxidation state [27] , [56] . Overall, benefiting the stabilizing enriched O V and low-valent active sites (Ru–O–Rh), the Rh-RuO 2 /G catalyst performs excellent activity and durability. Theoretical insights on intrinsic activity and stability DFT calculations were performed to understand the chemical origin of excellent OER activity and stability over Rh-RuO 2 /G. RuO 2 (110), (211), and (101) perfect (‘p’) surfaces, three dominant peaks in the XRD pattern (Fig. 2a ), were chosen as possible active surfaces. The defect RuO 2 surfaces (‘O V ’) and Rh doping RuO 2 surfaces (‘d’) were also calculated for comparison. Correspondingly, the ‘d-O V ’ denotes the defect RuO 2 surfaces with Rh doping. Based on previous studies [57] , [58] , three OER mechanisms were considered, as shown in Supplementary Fig. 14 , namely, AEM and two evolutionary lattice oxygen mediated mechanisms, LOM-OVSM and LOM-SMSM. For LOM-OVSM mechanism, a water molecule first deprotons to produce *OH at the O V site next to the doped Rh site, resulting in Ru–OH bond, followed by deprotonation and *O formation. Then, another water deprotons and produce an *OOH. Finally, as the final deprotonation occurs, an O 2 molecule can be evolved and desorbed from the surface, simultaneously reproducing the O V again. According to the scaling relations between the adsorption free energies (Supplementary Figs. 15– 17 ), the adsorption free energies of *OH and *OH_O V and *OH_SM are used as the primary descriptors of the reaction free energies ( ΔG ) of all elementary steps. Furthermore, the adsorption free energies of *O, *O_O V , and *OOH_SM are introduced as another dimension to build the two-dimensional activity maps of different mechanisms, as shown in Fig. 5a–c . DFT calculated free energy diagrams are shown in Supplementary Fig. 18 , where the activities (overpotentials) over different surfaces are compared. It is found that the *OOH formation limited its overall activity in the perfect RuO 2 and defect RuO 2 surfaces, while the potential-determining step of defect Rh-RuO 2 is the formation of *O (0.34 eV) by the synergistic effect of Rh doping and O V . Therefore, the activity of the examined catalysts is predicted to be defect Rh-RuO 2 > defect RuO 2 > perfect RuO 2 , with the distinctive mechanisms, namely, LOM-OVSM, LOM-OVSM, and AEM, respectively. A quantitative comparison between theoretical overpotentials and experimental ones exhibits a good correlation, which confirms our calculations and analysis above regarding the active site and reaction mechanism (Fig. 5d ). It is indicated that the OER over the d-O V 211 facet of the experimental Rh-RuO 2 /G samples is likely to follow the LOM-OVSM, which is attributed to the synergistic interaction of O V with the nearby metal site, consistent with the results observed by quasi in situ XPS. Fig. 5: DFT calculation of the OER reaction mechanism to elucidate intrinsic activity and stability of Rh-RuO 2 . a – c A two-dimensional activity map for AEM mechanism ( a ), LOM-OVSM mechanism ( b ), and LOM-SMSM ( c ) mechanism based on OER. The adsorption energies of *OH (*OH_O V or *OH_SM) and *O (*O_O V or *O_SM) are applied to be two independent descriptors. A 0.2 eV error bar is shown to describe the theoretical uncertainty. d Comparisons between calculated overpotential and experiment overpotential relationship. e A two-dimensional stability map for d and d-O V . f Charge density difference analysis for d and d-O V slab. Full size image As reported previously [59] , it is proposed that the stability loss of OER catalysts is induced by the dissolution of RuO 4 species; the catalyst is gradually deactivated in this process (see the proposed mechanism in Supplementary Fig. 19 ). To understand the stability of Rh-RuO 2 , the dissolution energy of RuO 4 species was calculated. The stability of various active sites is shown in Fig. 5e , where the blue area denotes better stability. Although the d-O V 211 facet of Rh-RuO 2 exhibits moderate stability, compared to d-O V 110 and d-O V 101, d-O V 211 should exhibit a dominant contribution to OER performance, considering both activity and stability. Furthermore, to interpret the activity and stability of d-O V 211, we compared the electronic structures of Rh-doped case and d-O V 211 based on the charge density difference analysis. As O V are introduced, the modified site (d-O V 211) becomes a better active center with lower electron density, resulting from the appropriate binding energy of reacting species, which is the fundamental reason for the improved activity of Rh-RuO 2 . In addition, as depicted in Fig. 5f , the electronic density on the surface Ru between d211 and d-O V 211 is comparable (1.74 vs. 1.71) based on Bader charge analysis, showing that the stability was not reduced. Hence, the observed OER stability can be understood well by DFT results. As for the contribution of RhO 2 for OER, the large-size RhO 2 nanocrystals can be excluded by the XRD pattern of Rh/G (Supplementary Fig. 5 ). DFT calculations were performed to investigate the contribution of OER activity from RhO x clusters as the adsorption energies are site- and size-dependent. Rh 6 O 6 and Rh 6 O 12 clusters were considered, supported on the most stable RuO 2 (101) facet, and two sites for all the clusters. Further, we considered both perfect and defective RuO 2 (101) as substrates. At some sites, the activity of RhO x clusters is indeed great (Supplementary Table 8 ). For instance, the sites of Rh 6 O 6 cluster on defect RuO 2 (101) substrate show similar overpotential (0.32 V vs. RHE) compared with the defect RuO 2 surfaces with Rh doping (0.34 V vs. RHE). Therefore, the contribution from the intrinsic activity of small RhO x clusters cannot be strictly ruled out [57] . It is noted that RhO x clusters should be dominated by high oxidation states, as the limited oxygen vacancies on pure RuO 2 under OER condition. In other words, the Rh 6 O 12 supported by perfect RuO 2 (101) should be the major case compared to the others, whose overpotentials are pretty large (1.67 V and 1.93 V vs. RHE). Besides, all the studied facets of Rh-RuO 2 are more stable compared to individual RhO 2 (Supplementary Table 10 ). By the combined analysis of experimental and computational results (both activity and stability), the Rh element should be primarily present as Rh-RuO 2 . In addition to the acidic OER performance, Rh-RuO 2 /G also performs impressive full water splitting catalytic performance with a cell voltage of 1.45 V and long-term stability in alkaline electrolyte, significantly exceeding RuO 2 /G and commercial RuO 2 (Supplementary Fig. 12 ). It is suggested that the intrinsic defect structure and rich active sites working together optimize the adsorption activation process of the intermediate to reduce the overpotential of the electrocatalytic reaction. Not only that, we leverage the OER electrocatalytic activity of Rh-RuO 2 /G as cathode catalysts in Li-O 2 battery (Supplementary Fig. 13 ), showing efficiently reduced charge overpotential of 0.27 V and long-term stability with a long cycle life of 4500 h, further illustrating the potential of this material in diversified energy catalysis and conversion systems. In summary, we demonstrate a synergetic regulation strategy of Rh doping and surface oxygen vacancies in stabilizing low-valent Ru of RuO 2 catalyst, arousing a LOM-OVSM pathway for impressive active and durable OER in harsh acidic media. Our stabilized Rh-RuO 2 /G catalyst shows a low overpotential of η 10 = 161 mV and long-term stability for 700 h at 50 mA cm −2 , surpassing most reported noble metal-based catalysts. It is validated that the presence of reversible oxygen vacancies improves the intrinsic activity and crystal structure stability under working potentials verified by quasi in situ / operando characterization techniques. DFT reveals that the Ru–O–Rh site with defect induces LOM-OVSM mechanism for extraordinary activity and durability. The formation of *O is the RDS of Rh-RuO 2 /G, breaking the AEM-limited reaction barrier (*OOH) of the conventional RuO 2 system. This work suggests new inspiration to design high-performance acidic OER catalysts and in-depth mechanistic analysis for practical application in PEM electrolyzers. Chemicals Ruthenium (III) chloride trihydrate (RuCl 3 ·3H 2 O), Rhodium (III) chloride (RhCl 3 ), and commercial RuO 2 were purchased from Aladdin Co., Ltd. The GO solution (6.2 mg ml −1 ) was synthesized via the modified Hummers’ method. Preparation of Rh-RuO 2 /G First, 5 ml GO solution (6.2 mg ml −1 ) was diluted with 26 ml water, then mixed with 15 mg RuCl 3 ·xH 2 O and 1 mg RhCl 3 to form a homogeneous solution. Further, the mixture was frozen with liquid nitrogen and vacuum freeze drying for 72 h. Finally, the as-obtained powder was annealed with air under 300 °C for 3 h, leading to the formation of Rh-RuO 2 /G. For comparison, RuO 2 /G nanosheets were synthesized according to a similar protocol without adding RhCl 3 ; Rh/G nanosheets were synthesized according to a similar protocol without adding RuCl 3 . Materials characterization XRD was performed by a SmartLab with Cu Kα radiation. SEM images were acquired on a JSM7900F. TEM, HRTEM, HAADF-STEM images, and elemental mapping images were detected by an HT7700 microscope and ARM300 microscope with spherical aberration corrector. AFM images were conducted on a MultiMode 3D. XPS spectra were recorded on Hermo Scientific K-Alpha. ICP-AES was measured in PerkinElmer Optima 7300DV for quantifying metal content in the catalysts. EPR was carried out on a Bruker A200 at 77 K. Raman spectroscopy was recorded by LabRAM HR 800 with an excitation laser of 532 nm. The N 2 sorption isotherms and Brunauer–Emmett–Teller (BET) surface areas were conducted by ASAP 2020 instrument at 77 K. H 2 -TPR experiments were performed with an AutoChem 2920 instrument. The XANES and EXAFS data were collected in the BL14W1 beamline of the Shanghai Synchrotron Radiation Facility (SSRF) under ambient air. EXAFS analysis, including calibration of the energy scale, correction of signal background, normalized signal intensity, and Fourier transform on k 2 -weighted EXAFS oscillations, was carried out on Athena software. Electrochemical measurements Electrochemical measurements were evaluated in 0.5 M H 2 SO 4 electrolyte (pH = 0.3) with a three-electrode configuration by a CHI 760E workstation. The cell contained a catalyst-modified glassy carbon electrode (GCE, 3 mm in diameter), Ag/AgCl filled with saturated KCl, and a graphite rod as the working electrode, the reference electrode, and the counter electrode, respectively. Furthermore, the well-dispersed catalyst loading on the GCE was ~0.45 mg cm −2 . LSV curves were carried out at 5 mV s −1 with 95% iR drop compensation. As for the durability test of chronopotentiometry, 40 μl catalyst ink (5 mg ml −1 ) was evenly scribbled on the surface of the titanium mesh, and the mass loading density of all samples in titanium mesh was ~1.25 mg cm −2 . Moreover, the same electrode fabrication method is used for water splitting in a two-electrode system. Potentials measured were converted to reversible hydrogen electrode (RHE) by the following equation: E (RHE) = E (Ag/AgCl) + 0.059 pH + 0.197. Quasi/in situ and operando characterizations XPS measurements were performed using the SPECS NAP-XPS instrument attached to the glove box through a vacuum channel. The Rh-RuO 2 /G catalysts subjected to OER reaction at a range of potentials (1.05–1.55 V vs. RHE) were transferred to the analysis chamber utilizing a vacuum channel for further XPS measurements. Operando DEMS with isotope labeling measurements were carried out in an electrochemical cell with a typical three-electrode system using the QAS 100 device (Linglu Instruments, Shanghai). The Rh-RuO 2 /G catalyst was labeled with 18 O isotopes by performing four times LSV cycles at 1.1–1.9 V (vs. RHE) with a scan rate of 5 mV s −1 in H 2 18 O aqueous sulfuric acid electrolyte. Meanwhile, the mass signals of different molecular weight gas products were recorded in real time. After cleaning the surface of electrodes with H 2 16 O, the same electrochemical and mass spectrometry were operated for 18 O-labeled Rh-RuO 2 /G catalyst in H 2 16 O aqueous sulfuric acid electrolyte. In situ Raman measurements were carried out in an in situ Raman cell equipped with a three-electrode system. Simultaneous acquisition of multipotential Raman spectra while catalyst OER procedure. Raman spectra were recorded by a LabRAM HR 800 Raman spectrometer with an excitation laser of 532 nm. Theoretical calculation methods All calculations were performed by Vienna Ab initio Simulation Package (VASP) [60] based on the DFT method, the generalized gradient approximation (GGA) [61] of the Perdew–Burke–Ernzerhof (PBE) [62] functional, and the projector-augmented wave (PAW) [63] , [64] with a cutoff of 450 eV were applied. The perfect RuO 2 (p), Rh-doped RuO 2 (d), and the defective systems (O V and d-O V ) were all studied. The (110), (101), and (211) surfaces were chosen, respectively, for modeling the facets that were observed experimentally for nanocrystalline rutile oxides [28] , [65] . 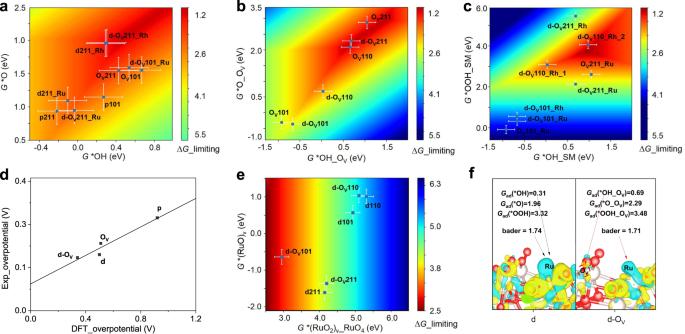Fig. 5: DFT calculation of the OER reaction mechanism to elucidate intrinsic activity and stability of Rh-RuO2. a–cA two-dimensional activity map for AEM mechanism (a), LOM-OVSM mechanism (b), and LOM-SMSM (c) mechanism based on OER. The adsorption energies of *OH (*OH_OVor *OH_SM) and *O (*O_OVor *O_SM) are applied to be two independent descriptors. A 0.2 eV error bar is shown to describe the theoretical uncertainty.dComparisons between calculated overpotential and experiment overpotential relationship.eA two-dimensional stability map for d and d-OV.fCharge density difference analysis for d and d-OVslab. In addition, the surface energy of the mixed phase with respect to pure metal phases and individual oxide phases were studied, respectively (Supplementary Table 5 and Table 10 ). Furthermore, the effect of different amounts of Rh incorporation on the stability was tested (Supplementary Table 6 ). The Monkhorst-Pack scheme with the k points of (3×2×1) and (2×3×1) were applied for the (110)/(211) and (100) surfaces, respectively. All fix the bottom half of the atoms during optimization. In addition, a 20 Å vacuum layer along the c -axis was used to eliminate the interactions of periodic images. Dipole corrections were applied to account for possible dipole interactions between unit cells. The convergence criteria for energy and force were set to 10 −4 eV and 0.03 eV Å −1 , respectively. In addition, spin-polarization was considered. All energies calculated by DFT are corrected to the temperature of 298 K. Computational hydrogen electrode approximation was used to implicitly describe the chemical potential of a (H + + e − ) pair. Theoretical activity and stability analysis The adsorption free energy of each intermediate was first calculated with reference to H 2 O(l) and H 2 (g). For example, the *OH is calculated as G (*OH) = E ad (*OH) + ZPE(*OH) − TS(*OH), where the G (*OH) was the adsorption free energy of intermediate *OH, the E ad (*OH) is the adsorption energy of *OH, the ZPE(*OH) is the zero-point energy of *OH, and the TS(*OH) is entropy correction, respectively (Supplementary Table 7 ). The scaling relationships of all adsorption free energies are shown in Supplementary Figs. 15– 17 . Then, the reaction energy (Δ G ) of each elementary step, such as *OH → *O + (H + + e − ), can be calculated as Δ G = G (*O) + G (H + + e − ) − G (*OH), where G (*O) is the adsorption energy of *O and G (H + + e − ) is the chemical potential of the proton and electron pair at 0 V vs. RHE calculated according to the computational hydrogen electrode [66] . G (H + + e − ) was a constant under a certain voltage, and G (*O) was linearly correlated with G (*OH). Therefore, Δ G was also linearly scaled with G (*OH). As a result, the Δ G as a linear function of G (*OH) can be obtained. More details can be found in our previous work [67] , [68] , [69] , [70] . Theoretical stability analysis As shown in Supplementary Fig. 19 , the theoretical stability of the electrode is described by the reaction free energy (Δ G limiting ) of the most thermodynamically difficult elementary step during the dissolution of ‘RuO 4 ’ species [59] .